The developmental basis of bat wing muscle By acquiring wings, bats are the only mammalian lineage to have achieved flight. To be capable of powered flight, they have unique muscles associated with their wing. However, the developmental origins of bat wing muscles, and the underlying molecular and cellular mechanisms are unknown. Here we report, first, that the wing muscles are derived from multiple myogenic sources with different embryonic origins, and second, that there is a spatiotemporal correlation between the outgrowth of wing membranes and the expansion of wing muscles into them. Together, these findings imply that the wing membrane itself may regulate the patterning of wing muscles. Last, through comparative gene expression analysis, we show Fgf10 signalling is uniquely activated in the primordia of wing membranes. Our results demonstrate how components of Fgf signalling are likely to be involved in the development and evolution of novel complex adaptive traits. Bats (order Chiroptera) acquired wings to become the only mammalian lineage with the ability of powered flight. They have adapted to various environments through tremendous variation on a basic single body plan and now constitute over 20% of extant mammalian species [1] , [2] . Recent molecular phylogenetic analysis supports the monophyly of bats, suggesting a single origin of powered flight in mammals [3] . It is almost universally accepted that bats evolved from small arboreal mammals [2] , [4] . However, to date there are no mammalian fossils of intermediate morphology linking bats to gliding or flightless ancestors [5] , implying the sudden appearance of this mammalian lineage with a unique body plan. The earliest known fossil bat, Onychonycteris finneyi , from the early Eocene was clearly capable of powered flight, possessing a forelimb that was morphologically similar to that of extant bats [6] . This has led some authors to hypothesize that bats achieved powered flight in a relatively short period of geological time, possibly through small changes in gene regulation during organogenesis [7] , [8] . However, the fossil record of bats is currently quite poor [9] , so there is still a possibility that transitional fossils may be discovered in the future. In that case, the evolution of the unique body plan of bats might be better explained by means of gradual processes, such as the divergence of many regulatory elements for several developmental control genes [10] . In any case, molecular and cellular mechanisms underlying the evolution of the bat wing remain poorly understood. In this paper we focused on the wing muscles—a synapomorphic character supporting the monophyly of bats [11] , [12] . Bats have an architecturally unique muscle complex called the occipito-pollicalis that extends along the anterior wing membrane (propatagium) and is necessary for powered flight ( Fig. 1a ) [13] . In addition, they possess sheets of muscles composed of the coraco-cutaneus, the humeropatagialis and the plagiopatagialis within the lateral wing membrane (plagiopatagium), and the uropatagialis within the interfemoral wing membrane (uropatagium) ( Fig. 1a ). These muscles are considered to have essential roles in controlling the shape of the wing and allowing the bats to fly [14] . Through detailed description of the ontogeny of wing muscles and their associated tissues in bat embryos, we have revealed that bat wing muscles are derived from multiple myogenic sources with different embryonic origins, and there is a spatiotemporal correlation between the outgrowth of wing membranes and the expansion of wing muscles into them. Furthermore, through comparative gene expression analysis, we found Fgf10 signalling is uniquely activated in the primordia of wing membranes and connective tissues within the membranes that may affect the architectural patterning of bat wing muscles. 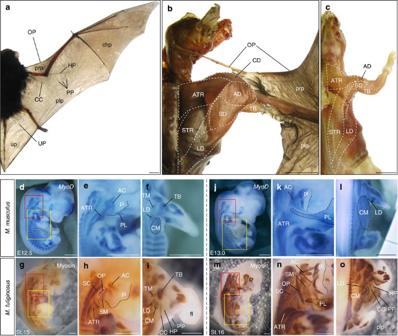Figure 1: Development of bat wing muscles. (a) Dorsal view of the wing of an adult bat (Miniopterus fuliginosus). (b,c) Comparison of muscle anatomy in bat and mouse. Note unique wing muscle called occipito-pollicalis (OP) that originates at occipital region of the head and enters into the propatagium (prp) in bat (b). (d–o) Comparison of pattern of muscle formation in mouse embryos (d–f,j–l) and bat embryos (g–i,m–o). (d) Lateral view of E12.5 mouse embryo. (e,f) Higher magnification of the red and yellow rectangles ind. (g) Stage 15 bat embryo. (h,i) Higher magnification of the rectangles ing. (j) E13.0 mouse embryo. (k,l) Higher magnification of the rectangles inj. (m) Stage 16 bat embryo. (n,o) Higher magnification of the rectangles inm. The acromiotrapezius (ATR) of mouse expands anteriorly almost covering the whole neck, so the splenius capitis (SC) and the sternomastoid (SM) located under ATR are not visible in these specimens. AC, auricularis; AD, acromiodeltoideus; CC, coraco-cutaneus; CD, clavodeltoideus; chp, chiropatagium; CM, cutaneus maximus; GM, gluteus maximus; HP, humeropatagialis; LD, latissimus dorsi; pi, pinna; PL, platysma; plp, plagiopatagium; PP, plagiopatagialis; STR, spinotrapezius; TB, triceps brachii; TM, teres major; UP, uropatagialis; up, uropatagium. Scale bars, 10 mm (a–c); 1 mm (d–o). Figure 1: Development of bat wing muscles. ( a ) Dorsal view of the wing of an adult bat ( Miniopterus fuliginosus ). ( b , c ) Comparison of muscle anatomy in bat and mouse. Note unique wing muscle called occipito-pollicalis (OP) that originates at occipital region of the head and enters into the propatagium (prp) in bat ( b ). ( d – o ) Comparison of pattern of muscle formation in mouse embryos ( d – f , j – l ) and bat embryos ( g – i , m – o ). ( d ) Lateral view of E12.5 mouse embryo. ( e , f ) Higher magnification of the red and yellow rectangles in d . ( g ) Stage 15 bat embryo. ( h , i ) Higher magnification of the rectangles in g . ( j ) E13.0 mouse embryo. ( k , l ) Higher magnification of the rectangles in j . ( m ) Stage 16 bat embryo. ( n , o ) Higher magnification of the rectangles in m . The acromiotrapezius (ATR) of mouse expands anteriorly almost covering the whole neck, so the splenius capitis (SC) and the sternomastoid (SM) located under ATR are not visible in these specimens. AC, auricularis; AD, acromiodeltoideus; CC, coraco-cutaneus; CD, clavodeltoideus; chp, chiropatagium; CM, cutaneus maximus; GM, gluteus maximus; HP, humeropatagialis; LD, latissimus dorsi; pi, pinna; PL, platysma; plp, plagiopatagium; PP, plagiopatagialis; STR, spinotrapezius; TB, triceps brachii; TM, teres major; UP, uropatagialis; up, uropatagium. Scale bars, 10 mm ( a – c ); 1 mm ( d – o ). Full size image Development of bat wing muscles As an initial step to understand the developmental origin of bat wing muscles, we described their ontogeny. The occipito-pollicalis forms from two spatially separated precursors: the proximal and distal elements. The former was first detected as a small muscle mass posterior to the muscle of the pinna (auricularis) and dorsal to the sternomastoid in bat embryos at stage 15 ( Fig. 1g ). The muscle expanded longitudinally at stage 16 ( Fig. 1m ). The latter was first recognized as a slender muscle mass within the already expanded propatagium at stage 17 ( Supplementary Fig. S1 ). The coraco-cutaneus, humeropatagialis and plagiopatagialis muscles were first recognized within the primordium of the plagiopatagium at stage 15 ( Fig. 1i ), and the muscular layer had further expanded in the tissue of the plagiopatagium at stage 16 ( Fig. 1o ). The uropatagialis first appeared as a sheet of muscle within the tissue between the tail and proximal part of the hind limb at stage 16 ( Supplementary Fig. S2 ). Innervation pattern and origin of bat wing muscles To identify the developmental origin and the homology of these muscles, we examined the innervation pattern, which has been used as a criterion for establishing muscle homology because of its close link to myogenesis [15] . Our analysis revealed that both proximal and distal elements of the occipito-pollicalis were solely innervated by cranial nerve VII (the facial nerve), as well as the auricularis and the platysma ( Fig. 2a ; Supplementary Fig. S1 ; Supplementary Movies ). This indicates the occipito-pollicalis associated with bat wings is derived from cranial paraxial mesoderm that later migrates into the second pharyngeal arch of the embryo. This is mostly consistent with results based on the dissection of adult bats [15] . The coraco-cutaneus and humeropatagialis within the plagiopatagium were innervated by spinal nerves that constitute the brachial plexus: cervical nerves 5–8 (C5–C8) and thoracic nerve 1 (T1) ( Fig. 2c ; Supplementary Movies ). This indicates these muscles share their developmental origin with muscles developed in the forelimb. The uropatagialis within the uropatagium is innervated by a group of spinal nerves that constitute the lumbar and sacral plexuses, especially by the nerve branch that topologically corresponds to the branch innervating the anteromedial part of the semitendinosus in mouse embryos ( Supplementary Fig. S2 ; Supplementary Movies ). This indicates the muscle shares a developmental origin with skeletal muscles of the hind limb. As a whole, these data suggest that multiple populations of muscle precursors with different ontogenetic origins were involved in building the bat wing. 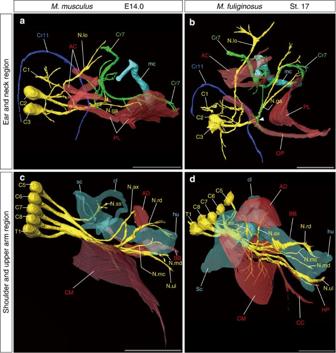Figure 2: Innervation pattern of bat wing muscles. (a) Innervation of the muscles associated with the ear and the neck of mouse embryo at E14.0 (right side, dorsolateral view). (b) Innervation of the proximal element of the occipito-pollicalis associated with the propatagium of bat embryo at stage 17. Meckel’s cartilage (mc) is used as the landmark to show the location of the lower jaw of the embryos. The occipito-pollicalis is innervated by a branch of cranial nerve VII (arrowhead inb), implying close ontogenetic relationship between the posterior part of the platysma of mouse and the occipito-pollicalis of bat. Cranial nerve XI (the accessory nerve) of bat embryos does not innervate the occipito-pollicalis but does innervate the trapezius, sternomastoid and cleidomastoid (not shown for simplicity) as in mouse embryo. (c) Innervation of skeletal muscles in shoulder and upper arm regions in mouse embryo at E14.0 (right side, dorsolateral view). (d) Innervation of the coraco-cutaneus (CC) and humeropatagialis (HP) muscle complex associated with the plagiopatagium in bat embryo at stage 17. The acromiodeltoideus (AD) and the biceps brachii (BB) are shown as landmarks. Two muscles developed within the plagiopatagium of bats are innervated by cervical and thoracic nerves that constitute the brachial plexus, implying these muscles share developmental origin with the muscles of the forelimb. cl, primordium of clavicle; Cr7, branch of cranial nerve VII (the facial nerve); Cr11, branch of cranial nerve XI (the accessory nerve); C1, ganglion of cervical nerve 1; C2, ganglion of cervical nerve 2; C3, ganglion of cervical nerve 3; C5, ganglion of cervical nerve 5; C6, ganglion of cervical nerve 6; C7, ganglion of cervical nerve 7; C8, ganglion of cervical nerve 8; hu, humerus or its primordium; mc, Meckel's cartilage; N.ax, axillary nerve; N.Ga, great auricular nerve; N.lo, lesser occipital nerve; N.md, median nerve; N.mc, musculoctaneus nerve; N. pr, perineal nerve; N.rd, radial nerve; N.ss, suplascapular nerve; N.ul, ulnar nerve; sc, primordium of scapula; T1, ganglion of thoracic nerve 1. Scale bars, 1 mm. Figure 2: Innervation pattern of bat wing muscles. ( a ) Innervation of the muscles associated with the ear and the neck of mouse embryo at E14.0 (right side, dorsolateral view). ( b ) Innervation of the proximal element of the occipito-pollicalis associated with the propatagium of bat embryo at stage 17. Meckel’s cartilage (mc) is used as the landmark to show the location of the lower jaw of the embryos. The occipito-pollicalis is innervated by a branch of cranial nerve VII (arrowhead in b ), implying close ontogenetic relationship between the posterior part of the platysma of mouse and the occipito-pollicalis of bat. Cranial nerve XI (the accessory nerve) of bat embryos does not innervate the occipito-pollicalis but does innervate the trapezius, sternomastoid and cleidomastoid (not shown for simplicity) as in mouse embryo. ( c ) Innervation of skeletal muscles in shoulder and upper arm regions in mouse embryo at E14.0 (right side, dorsolateral view). ( d ) Innervation of the coraco-cutaneus (CC) and humeropatagialis (HP) muscle complex associated with the plagiopatagium in bat embryo at stage 17. The acromiodeltoideus (AD) and the biceps brachii (BB) are shown as landmarks. Two muscles developed within the plagiopatagium of bats are innervated by cervical and thoracic nerves that constitute the brachial plexus, implying these muscles share developmental origin with the muscles of the forelimb. cl, primordium of clavicle; Cr7, branch of cranial nerve VII (the facial nerve); Cr11, branch of cranial nerve XI (the accessory nerve); C1, ganglion of cervical nerve 1; C2, ganglion of cervical nerve 2; C3, ganglion of cervical nerve 3; C5, ganglion of cervical nerve 5; C6, ganglion of cervical nerve 6; C7, ganglion of cervical nerve 7; C8, ganglion of cervical nerve 8; hu, humerus or its primordium; mc, Meckel's cartilage; N.ax, axillary nerve; N.Ga, great auricular nerve; N.lo, lesser occipital nerve; N.md, median nerve; N.mc, musculoctaneus nerve; N. pr, perineal nerve; N.rd, radial nerve; N.ss, suplascapular nerve; N.ul, ulnar nerve; sc, primordium of scapula; T1, ganglion of thoracic nerve 1. Scale bars, 1 mm. Full size image Outgrowth of wing membranes and expansion of wing muscles Through inspection of the pattern of wing muscle development, we found a spatiotemporal correlation between the outgrowth of wing membranes and expansion of the mass of wing muscle precursors towards the membranes. In the neck/shoulder region of bat embryos, the primordium of the occipito-pollicalis expanded in a posterior–lateral direction towards the growing propatagium ( Fig. 3a ; Supplementary Fig. S3 ). We confirmed the coraco-cutaneus and humeropatagialis complex originated from migrating muscle precursors that delaminated from the ventrolateral lips of dermomyotome of somites at the limb level ( Supplementary Fig. S4 ). At stage 14L, the wing muscle complex shared a common muscle progenitor with the cutaneus maximus, which expanded in a postero-dorsal direction in later stages ( Fig. 3e ). Interestingly, the wing muscle complex was separated from the cutaneus maximus progenitor by a population of non-muscle ( Lbx1 negative) connective tissues and expanded in a posterior–lateral direction towards growing plagiopatagium in subsequent embryonic stages ( Fig. 3f ; supplementary Fig. S5 ). A similar pattern of muscle development also was observed in the uropatagium ( Supplementary Fig. S2 ). These data suggest that the tissue of the wing membrane likely has an important role in determining the architectural pattern of bat wing muscles. 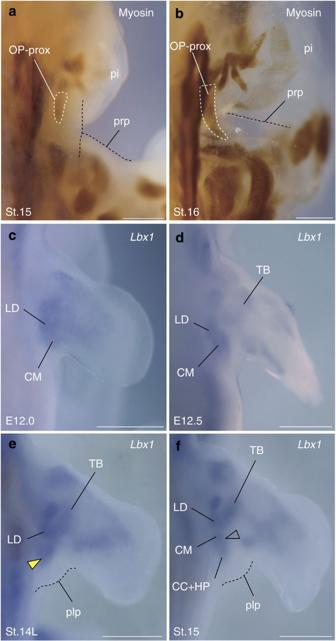Figure 3: Spatiotemporal correlation between outgrowth of wing membranes and expansion of wing muscles. (a,b) Dorsal view of neck and shoulder regions of bat embryos at stage 15 and stage 16, respectively. In these periods of bat embryogenesis, the propatagium (prp) grows anterolaterally and the precursor of the proximal element of the occipito-pollicais (OP-prox) expands in a posterolateral direction and begins to enter into the membrane. (c,d) Dorsal view of the forelimb region of mouse embryos at E12.0 and E12.5, respectively. (e,f) Dorsal view of the forelimb region of bat embryos at stage 14L and stage 15, respectively. Precursors of limb muscles in these embryos were labelled byin situhybridization withLbx1probe. Yellow arrowhead ineindicates the muscle mass that contains the precursors of cutaneus maximus (CM), coraco-cutaneus (CC) and humeropatagialis (HP). The muscle complex is subdivided into two populations at the middle point (open arrowhead): anteromedially-located CM precursor and posterolaterally located precursor for CC and HP (CC+HP) in subsequent stage. The posterior tip of the latter directs towards the primordium of the plagiopatagium that grows posterolaterally. LD, latissimus dorsi; TB, triceps brachii. Scale bars, 0.5 mm. Figure 3: Spatiotemporal correlation between outgrowth of wing membranes and expansion of wing muscles. ( a , b ) Dorsal view of neck and shoulder regions of bat embryos at stage 15 and stage 16, respectively. In these periods of bat embryogenesis, the propatagium (prp) grows anterolaterally and the precursor of the proximal element of the occipito-pollicais (OP-prox) expands in a posterolateral direction and begins to enter into the membrane. ( c , d ) Dorsal view of the forelimb region of mouse embryos at E12.0 and E12.5, respectively. ( e , f ) Dorsal view of the forelimb region of bat embryos at stage 14L and stage 15, respectively. Precursors of limb muscles in these embryos were labelled by in situ hybridization with Lbx1 probe. Yellow arrowhead in e indicates the muscle mass that contains the precursors of cutaneus maximus (CM), coraco-cutaneus (CC) and humeropatagialis (HP). The muscle complex is subdivided into two populations at the middle point (open arrowhead): anteromedially-located CM precursor and posterolaterally located precursor for CC and HP (CC+HP) in subsequent stage. The posterior tip of the latter directs towards the primordium of the plagiopatagium that grows posterolaterally. LD, latissimus dorsi; TB, triceps brachii. Scale bars, 0.5 mm. Full size image Fgf10 signalling in bat wing development To date, the molecular mechanism underlying the development of the bat wing membrane has not been understood, with the exception of one report that the modulation of Bmp and Fgf signalling has a role in blocking apoptosis of interdigital tissue to make the interdigital wing membrane (chiropatagium) [16] . Through comparative expression analysis of the genes that are known to regulate limb morphogenesis, we found Fgf10 signalling is likely involved in wing membrane development and patterning of the wing muscles. As reported in murine embryogenesis [17] , Fgf10 was expressed at the otic vesicle, pharyngeal arches and limb mesenchyme, as well as lateral plate mesoderm of the flank region of bat embryos at stage 13 ( Fig. 4a–c ). Interestingly, Fgf10 continued to be expressed in the lateral plate-derived mesenchyme at the anterior-proximal part of the forelimb, flank and posterior-proximal part of hind limb of bat embryos at stage 13L and 14 ( Figs 4d,f and 5a–c ; Supplementary Fig. S2 ), although expression of Fgf10 ceased in corresponding tissues of stage-matched mouse, marsupial opossum and chick embryos [17] , [18] , [19] . We also examined expression of Fgfr2IIIb that encodes the receptor of Fgf10 in bat embryos, and detected its expression in epidermis over the flank region of Fgf10 -expressing lateral plate mesoderm, as well as in epidermis of the limb buds and lateral plate mesoderm anterior to the forelimb bud at stage 13L ( Fig. 4e ). Concordant with a previous report [20] , Fgf8 was not expressed in the primordia of pro-, plagio- and uropatagium throughout embryogenesis, but only expressed in the apical ectodermal ridge (AER) postcranially ( Fig. 4h ). These results indicate that Fgf10 signalling is activated in the embryonic tissues where future wing membranes develop. 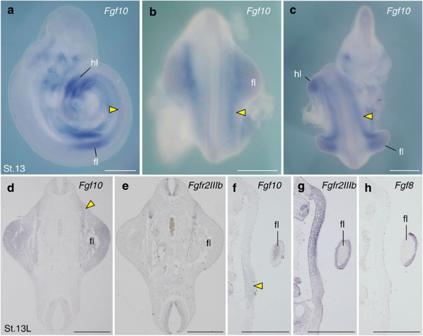Figure 4: Unique expression ofFgf10at the domain where future wing membranes develop. (a–c) Expression ofFgf10in bat embryo at stage 13. (a) Lateral view. (b) Dorsal view focusing on the forelimb bud (fl). (c) Frontal view focusing on the interlimb region.Fgf10is expressed in the lateral plate mesoderm of the interlimb level (yellow arrowheads ina,bandc), as well as in the lateral plate-derived mesenchyme of both forelimb and hind limb (hl) buds. (d,e) Sectionin situhybridization ofFgf10(d) andFgfr2IIIb(e) in horizontal sections of the forelimb region of bat embryo at stage 13L. Cranial side of the embryo is oriented to the top. NoteFgf10is expressed in the anterior domain of the forelimb buds where the primordium of propatagium is developed later (yellow arrowhead ind). Expression ofFgfr2IIIbis detected at the epidermis over theFgf10-positive forelimb mesenchyme, as well as in the mesenchyme anterior to the forelimb bud where expression ofFgf10is also detected. (f–h) Sectionin situhybridization ofFgf10(f),Fgfr2IIIb(g) andFgf8(h) in horizontal sections focusing on the lateral plate mesoderm at the interlimb level of the same embryo. Cranial side of the embryo is oriented to the top. Unique expression ofFgf10in lateral plate mesoderm at the interlimb level still remains in this stage (yellow arrowhead inf). Expression ofFgfr2IIIbis detected at the epidermis over theFgf10-positive flank mesenchyme and the forelimb bud, as well as in the lateral plate mesoderm anterior to the forelimb bud. Expression ofFgf8is only detected at the apical ectodermal ridge of the forelimb bud. Scale bars, 0.5 mm. Figure 4: Unique expression of Fgf10 at the domain where future wing membranes develop. ( a – c ) Expression of Fgf10 in bat embryo at stage 13. ( a ) Lateral view. ( b ) Dorsal view focusing on the forelimb bud (fl). ( c ) Frontal view focusing on the interlimb region. Fgf10 is expressed in the lateral plate mesoderm of the interlimb level (yellow arrowheads in a , b and c ), as well as in the lateral plate-derived mesenchyme of both forelimb and hind limb (hl) buds. ( d , e ) Section in situ hybridization of Fgf10 ( d ) and Fgfr2IIIb ( e ) in horizontal sections of the forelimb region of bat embryo at stage 13L. Cranial side of the embryo is oriented to the top. Note Fgf10 is expressed in the anterior domain of the forelimb buds where the primordium of propatagium is developed later (yellow arrowhead in d ). Expression of Fgfr2IIIb is detected at the epidermis over the Fgf10 -positive forelimb mesenchyme, as well as in the mesenchyme anterior to the forelimb bud where expression of Fgf10 is also detected. ( f – h ) Section in situ hybridization of Fgf10 ( f ), Fgfr2IIIb ( g ) and Fgf8 ( h ) in horizontal sections focusing on the lateral plate mesoderm at the interlimb level of the same embryo. Cranial side of the embryo is oriented to the top. Unique expression of Fgf10 in lateral plate mesoderm at the interlimb level still remains in this stage (yellow arrowhead in f ). Expression of Fgfr2IIIb is detected at the epidermis over the Fgf10 -positive flank mesenchyme and the forelimb bud, as well as in the lateral plate mesoderm anterior to the forelimb bud. Expression of Fgf8 is only detected at the apical ectodermal ridge of the forelimb bud. Scale bars, 0.5 mm. 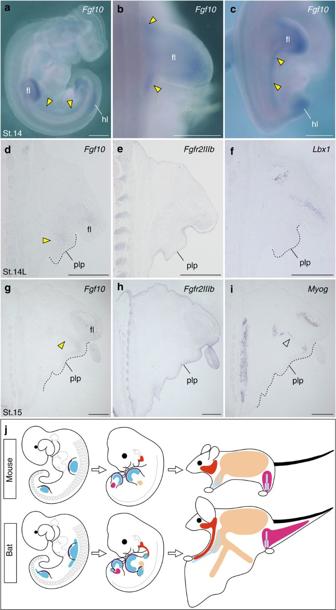Figure 5: Unique activation of Fgf10 signalling in wing membrane tissues. (a–c) Expression ofFgf10in bat embryo at stage 14. Unique expression ofFgf10is detected in the domains where future wing membranes develop (yellow arrowheads). (d–i) Sectionin situhybridization in the forelimb (fl) and plagiopatagium (plp) tissues of bat embryo at stage 14L (d–f) and stage 15 (g–i).Fgf10is expressed in the mesenchyme inside the primordium of the plagiopatagium (yellow arrowheads) and its receptor gene,Fgfr2IIIb, is expressed in the epidermis that covers the forelimb and the plagiopatagium. Muscular tissue is not detected inside the primordium of plagiopatagium until stage 15 (f,i). (j) Schematic illustration for bat wing muscle evolution. In limb bud-stage, expression domain ofFgf10(blue) is expanded into the lateral plate mesoderm where future wing membranes develop. In these domains, Fgf10 signalling may regulate the outgrowth of wing membrane and the patterning of the skeletal muscles to build wing muscles. Purple,Fgf8expression in the AER. Red, the second pharyngeal arch-derived muscle progenitor. Orange, the muscle progenitor derived from migrating muscle precursors (MMPs) at forelimb level. Magenta, the muscle progenitor derived from MMPs at hind limb level. Right blue, stylopod and zeugopod elements of the limb skeleton. Scale bars, 0.5 mm. Full size image Figure 5: Unique activation of Fgf10 signalling in wing membrane tissues. ( a – c ) Expression of Fgf10 in bat embryo at stage 14. Unique expression of Fgf10 is detected in the domains where future wing membranes develop (yellow arrowheads). ( d – i ) Section in situ hybridization in the forelimb (fl) and plagiopatagium (plp) tissues of bat embryo at stage 14L ( d – f ) and stage 15 ( g – i ). Fgf10 is expressed in the mesenchyme inside the primordium of the plagiopatagium (yellow arrowheads) and its receptor gene, Fgfr2IIIb , is expressed in the epidermis that covers the forelimb and the plagiopatagium. Muscular tissue is not detected inside the primordium of plagiopatagium until stage 15 ( f , i ). ( j ) Schematic illustration for bat wing muscle evolution. In limb bud-stage, expression domain of Fgf10 (blue) is expanded into the lateral plate mesoderm where future wing membranes develop. In these domains, Fgf10 signalling may regulate the outgrowth of wing membrane and the patterning of the skeletal muscles to build wing muscles. Purple, Fgf8 expression in the AER. Red, the second pharyngeal arch-derived muscle progenitor. Orange, the muscle progenitor derived from migrating muscle precursors (MMPs) at forelimb level. Magenta, the muscle progenitor derived from MMPs at hind limb level. Right blue, stylopod and zeugopod elements of the limb skeleton. Scale bars, 0.5 mm. Full size image In bat embryos at stage 14L the primordium of plagiopatagium appeared posterior to the forelimb as a bud-like structure. We detected Fgf10 in the mesenchyme that populates in the primordium of plagiopatagium as well as in the mesenchyme of the forelimb ( Fig. 5d ; Supplementary Fig. S6 ). Fgfr2IIIb also was expressed in the epidermis over the forelimb and the primordium of plagiopatagium ( Fig. 5e ). At this period of bat embryogenesis, we did not observe myocytes that express lineage-specific markers such as Pax3 and Lbx1 inside the primordium of plagiopatagium ( Fig. 5f ; Supplementary Fig. S6 ). Furthermore, Tcf4 , which is known as a good marker for lateral plate-derived limb connective tissue and regulates the spatial pattern of limb muscles [21] , [22] , was not expressed in the mesenchyme within the plagiopatagium ( Supplementary Fig. S6 ). In the subsequent embryonic stage, where the precursor of the coraco-cutaneus and humeropatagialis complex starts to populate inside the plagioptagium, expression of Fgf10 was restricted to the connective tissue in close proximity to these wing muscles ( Fig. 5g ; Supplementary Fig. S6 ). We observed a similar pattern of Fgf10 expression in propatagium and uropatagium as well ( Supplementary Figs S2 and S7 ). In vertebrates, skeletal muscles which form in the head, trunk and limbs are patterned by extrinsic cues from surrounding tissues to adopt specific arrangements of muscle fibres in the adult form [23] , [24] , [25] , [26] , [27] , [28] , [29] , [30] , [31] . For example, somite-derived limb muscle precursor cells migrate into the limb bud which is filled with lateral plate-derived connective tissue. There, the muscles are extrinsically patterned by the connective tissues in later embryonic stages [32] , [33] . In bat embryogenesis, we observed a spatiotemporal correlation between the outgrowth of wing membranes and expansion of the mass of wing muscle precursors towards the membranes. The mass of all the wing muscle precursors we examined consistently expanded towards the growing wing membranes. The wing muscle precursors did not expand into other directions within the embryonic body nor stop their expansion around the domain where they originated. This suggests that the mode of bat wing muscle patterning resembles that of limb muscle patterning in which the limb bud filled with lateral plate-derived connective tissue dictates the patterning of the muscles migrated from the somites. On the basis of these observations, it appears reasonable to regard the wing membranes as a potential candidate tissue for patterning of the wing muscles. To obtain direct evidence that the wing membranes regulate patterning of the bat wing muscles, experimental approaches such as heterotopic transplantation of bat wing membrane tissues into ‘non-wing’ domains of mammalian embryos will be helpful. Through gene expression analysis in bat embryos, we observed Fgf8 expression in the AER of the limb and the absence of its expression in the tissue of all wing membranes we examined. Instead, we observed expression of Fgf10 not only in limb mesenchyme but also in the mesenchyme of the wing membrane primordia. Furthermore, expression of the gene encoding the receptor of Fgf10, Fgfr2IIIb , was detected in the overlaying epidermis and some populations of the underlying mesenchyme of the wing membrane primordia and in the limb epidermis, including the AER. In vertebrates, maintenance of proximodistal outgrowth of the embryonic limbs requires Fgf10 in the mesenchyme to activate Fgf8 in the AER, which in turn promotes mesenchymal outgrowth [18] , [34] , [35] , [36] . It appears that the outgrowths of the anterior, lateral and interfemoral wing membranes formed in bat embryos are achieved by a molecular mechanism that is partly different from that regulating the outgrowth of the limb. In terms of the mode of the tissue outgrowth, the primordia of these wing membranes more closely resemble other types of epithelial appendages such as feather buds in birds, secondary palate in mammals and external genitalia where Fgf10 signalling regulates their outgrowth [37] , [38] , [39] . As mentioned above, in principle, the architectural pattern of skeletal muscles is determined extrinsically by surrounding muscle connective tissue in vertebrate embryos. It has been reported that Tcf4 , a downstream effecter of canonical Wnt signalling that has pivotal roles in limb development, is expressed in lateral plate-derived limb connective tissue and regulates patterning of somite-derived limb muscles [21] , [22] . Therefore, we focused on this gene and examined its expression pattern in bat embryos. Intriguingly, expression of Tcf4 is detected in limb connective tissue, as in chicken and mouse embryos, but not in connective tissue within the wing membranes. Instead, we observed continued expression of Fgf10 in connective tissue within the wing membranes. Showing analogy with the spatiotemporal pattern of Tcf4 expression in the limbs, Fgf10 expression was detected in connective tissue of the nascent plagiopatagium and its expression preceded the entering of wing muscles into the membrane. In later stage embryos, expression domain of Fgf10 was restricted in the connective tissue adjacent to the wing muscles. Such spatiotemporal correlations between Fgf10 expression and the development of wing muscles were observed in the propatagium and uropatagium, as well. On the basis of the results of our minute description of bat wing morphogenesis, we speculate that Fgf10 may be a key molecule involved in the process of wing muscle patterning, as Tcf4 is in limb muscle patterning. Although molecular mechanisms controlling the organization of skeletal muscle in space during vertebrate development are not fully understood, signalling molecules secreted from non-myogenic mesenchyme or muscle connective tissue, as well as cell adhesion molecules localized at the cell membrane of muscle connective tissue, potentially affect the architectural pattern of muscles [21] , [22] , [30] , [40] , [41] , [42] , [43] , [44] , [45] , [46] , [47] , [48] . In tongue morphogenesis, cranial neural crest-derived tongue muscle connective tissue is required for organizing occipital somite-derived tongue muscle cells [49] . In this process, Fgf10 secreted from the surrounding muscle connective tissue possibly controls myogenic cell proliferation and potentially influences the organization of tongue muscle [49] . Fgf10 signal-mediated cell–cell interactions involved in other developmental events [50] , [51] , [52] also may contribute to the formation of unique wing muscles in bats. To uncover the role of Fgf10 in bat wing morphogenesis, functional analysis of this gene in bat embryos should be performed in the future. For the evolution of the flight apparatus in bats, we suppose that a two-step developmental mechanism was important ( Fig. 5j ). The first step is the establishment of the field for wing membrane formation possibly achieved by spatially unique activation of Fgf10 signalling in early stage bat embryos. The second step is the alteration of skeletal muscle pattern, perhaps driven by connective tissue filling the wing membranes, to make unique wing muscles. In bat embryogenesis, the outgrowth of wing membranes and wing myogenesis precede the elongation of zeugopodial and autopodial skeletons of the forelimb and retention of the tissue that gives rise to the chiropatagium, other vital events for bats to achieve powered flight. It would be interesting to further investigate how unique activation of Fgf10 signalling in wing membrane progenitors influences these upcoming embryonic events, as well as to identify the molecular basis which allows the novel anterior–posterior expanded Fgf10 expression we observed in non-limb lateral plate mesoderm of bat embryos. Primitive bat species such as Onychonycteris and Icaronycteris index had well-developed wings, implying that they were capable of powered flight [6] . Although the soft tissue anatomy of these fossil species is not well understood, the impression of wing membranes on some fossils indicates the presence of wing muscles in these animals [13] . Therefore, the developmental programme that mobilizes adjacent muscular tissues for the precursors of the wing membranes might have been adopted in the initial phase of chiropteran evolution, in parallel with the acquisition of the wing itself. Furthermore, recent molecular phylogeny of extant bat species clearly identifies two major lineages within the order—suborders Yinpterochiroptera and Yangochiroptera [2] , [53] , [54] . In the present study, we revealed that the occipito-pollicalis of Miniopterus fuliginosus (family Miniopteridae), which is a member of Yangochiroptera, is solely innervated by cranial nerve VII. According to previous studies [13] , [15] , the muscle complex of Pteropus (family Pteropodidae), which belongs to Yinpterochiroptera, is innervated by not only cranial nerve VII but also cervical nerves. Also, in contrast to the simple organization of the occipito-pollicalis in Miniopterus , that in Pteropus is reportedly more complex, composed of several muscle bellies [13] , [15] . We predict that the more complicated organization and innervation patterns of the occipito-pollicalis seen in pteropodid bats were brought about by the acquisition of unidentified novel developmental programs for establishing such anatomical features after they diverged from the common ancestor of Yangochiroptera or other lineages of Yinpterochiroptera. To better understand the developmental basis of bat wing muscle evolution, sampling embryos from a variety of chiropteran lineages, both Yinpterochiroptera and Yangochiroptera, and comparing their development will be necessary. Sample collection and staging of embryos Adult female Pipistrellus abramus (family Vespertilionidae) were captured in Kyoto prefecture, Japan, during the breeding seasons of 2005, 2006, 2008 and 2010. Adult female Miniopterus fuliginosus (family Miniopteridae) were collected in Wakayama prefecture, Japan, during the breeding seasons of 2009 and 2011. These animals were brought to the laboratory and killed after anesthetization by exposure to diethyl ether. The uteri were removed from the abdominal cavity of the animals and transferred to Petri dishes filled with 0.1 M PBS on ice. The walls of the uteri were cut open to remove the embryos, and then the embryos were excised with forceps from the surrounding extraembryonic membranes. Pregnant females of wild-type mice (ICR) were purchased commercially and embryos were sampled following standard protocol. Staging of bat embryos was as per previous studies [55] , [56] . Comparison of embryos between bats and mice was performed following the method of a previous study [56] . All animal experiments were approved by the University of Tsukuba Committee for Animal Care. Cloning of genes Total RNA was extracted from embryos using ISOGEN reagent (NIPPON GENE CO., LTD). RT–PCR was performed to amplify fragments of Pipistrellus Hgf and Pax3 , and Miniopterus c-Met, Fgfr2IIIb , Fgf10 , Lbx1 , Myogenin ( Myog ) and Tcf4 messenger RNA using primer sets that are available upon request. These fragments were isolated using the pGEM T-easy vector systems (Promega) or TOPO TA cloning kit (Invitrogen) and sequenced using an ABI 3130 sequencer (Applied Biosystems). To identify the orthologous genes of the isolated fragments, comparable sequence data were surveyed using a BLAST search, and phylogenetic trees with neighbour joining method were constructed after sequence alignment using the CLUSTALX software. All new DNA sequence data were deposited in the DDBJ database (AB761037, AB761038, AB761039, AB761040, AB761041, AB761042, AB761043 and AB761044). Gene expression analysis After fixing embryos in 4% paraformaldehyde (PFA), whole-mount in situ hybridization of bat and mouse embryos was conducted following a standard protocol [57] . For section in situ hybridization, embryos were fixed in 4% PFA, dehydrated using a methanol series, placed in xylene, embedded in paraffin and sliced with a microtome. Serial sections were hybridized with digoxigenin-labelled riboprobes as described in Neubüser et al. [58] with slight modifications. To detect expression of Lbx1 and Pax3 genes in mouse tissues, antisense RNA riboprobes constructed from complementary DNA sequences of bats were used. To detect expression of Fgf8 genes in bat tissues, RNA probe of mouse was used following the method of Weatherbee et al. [16] Generally, hetero-specific RNA probes easily hybridize with the transcripts among mammalian lineages, because of the low level of nucleotide sequence variation in the protein-coding regions of genes [57] , [59] . To confirm the expression pattern of each gene, two to four individual bat embryos were analysed for each stage. Muscle and nerve staining To visualize skeletal muscles and peripheral nerves whose motor branches innervate skeletal muscles in embryogenesis, whole-mount immunohistochemistry of anti-skeletal muscle myosin (MF20, DSHB) and anti-neurofilament (3A10, DSHB) antibodies were conducted following a standard protocol [60] . To confirm the localization pattern of myosin protein, two to four individual bat embryos were analysed for each stage. As MF20-stained mouse embryos tended to have non-specific background signals, possibly due to the reaction of secondary antibody against endogenous mouse IgG, whole-mount in situ hybridization of MyoD that continues to be expressed even in differentiated skeletal muscles of late stage embryos was alternatively used for muscle visualization in mouse embryos. Analysis of muscle innervation pattern The embryos were fixed with Serra’s fixative for 24 h, dehydrated using an ethanol series, placed in xylene, embedded in paraffin and sliced at a thickness of 12 μm. After deparaffinization of the sliced sections, immunohistochemistry of anti-acetylated tubulin (6-11B-1, SIGMA) monoclonal antibody was carried out to label nerve tissues. Subsequently, cell nuclei were stained with haematoxylin to distinguish muscular tissues from other tissues morphologically. Sections were photographed with a digital camera (VB-6010, KEYENCE) mounted on a dissection microscope (AZ100, Nikon). Amira 5.0 software was used to digitally reconstruct the sectioned and stained embryos in three dimensions, following the manufacturer’s instructions. How to cite this article: Tokita, M. et al. The developmental basis of bat wing muscle. Nat. Commun . 3:1302 doi: 10.1038/ncomms2298 (2012).